Vapor–liquid–solid growth of large-area multilayer hexagonal boron nitride on dielectric substrates Multilayer hexagonal boron nitride ( h -BN) is highly desirable as a dielectric substrate for the fabrication of two-dimensional (2D) electronic and optoelectronic devices. However, the controllable synthesis of multilayer h -BN in large areas is still limited in terms of crystallinity, thickness and stacking order. Here, we report a vapor–liquid–solid growth (VLSG) method to achieve uniform multilayer h -BN by using a molten Fe 82 B 18 alloy and N 2 as reactants. Liquid Fe 82 B 18 not only supplies boron but also continuously dissociates nitrogen atoms from the N 2 vapor to support direct h -BN growth on a sapphire substrate; therefore, the VLSG method delivers high-quality h -BN multilayers with a controllable thickness. Further investigation of the phase evolution of the Fe-B-N system reveals that isothermal segregation dominates the growth of the h -BN. The approach herein demonstrates the feasibility for large-area fabrication of van der Waals 2D materials and heterostructures. Recently, two-dimensional (2D) materials have received considerable attention as promising candidates for next-generation electronic and optoelectronic devices. However, they are very sensitive to their surroundings due to their 2D nature [1] , [2] . Hexagonal boron nitride ( h -BN), a typical dielectric substrate, could maintain the intrinsic properties of other 2D materials due to its atomic flatness and the absence of dangling bonds and charge impurities on its surface [3] , [4] , [5] . Extensive research has shown the outstanding performance of multilayer h -BN as a substrate in electronic devices made from 2D materials [1] , [4] . Therefore, the fabrication of high-quality h -BN over a large area provides promise for its application in 2D electronics and optoelectronics [6] , [7] , [8] , [9] . Through mechanical exfoliation [10] , high-quality multilayer h -BN flakes can be obtained from bulk h -BN crystals, which are typically synthesized by a metal-B-N solvent-assisted method under extreme temperatures (1500−1750 °C) and pressures (4.0−5.5 GPa) [11] . Limitations on the control of the lateral size and thickness prevent exfoliated h -BN from applications that require scaling. Therefore, much effort has been devoted to the mass production of large-area multilayer h- BN films. Currently, chemical vapor deposition (CVD) is a very successful method to grow h -BN on metals and alloys at relatively low cost [12] , [13] , [14] , [15] , [16] , [17] , [18] , [19] . However, catalytic effects always yield thin h -BN films, e.g., a thickness of a few layers (<10 layers), which could not efficiently protect electronic 2D crystals from the disturbance in their surroundings. The existing fabrication approaches use flammable and toxic chemicals, including borazine (B 3 N 3 H 6 ) 16 , or complicated chemicals, such as ammonia borane (H 3 NBH 3 ) [20] , as reactive precursors. In addition, the wet transfer process from metallic surfaces to target substrates would probably degrade the quality of the h -BN and then limit its application in microelectronics. We also noticed that there have been several reports about the direct synthesis of h -BN films on dielectric substrates [21] , [22] , but the low thickness control and high crystallinity of h -BN films are issues that remain elusive [21] , [22] , [23] , [24] . In this study, we demonstrated a vapor–liquid–solid growth (VLSG) method to fabricate high-quality multilayer h -BN films on (0001) sapphire substrates using an Fe 82 B 18 alloy and N 2 as reactants. The melting point of the Fe 82 B 18 (~1180 °C) is lower than that of most catalytic metal-B alloys. Besides, compared to commonly used NH 3 , N 2 is a safer choice and would be friendly to environment. The VLSG, first proposed by Wagner in 1964, is widely used for one-dimensional crystal growth [25] , [26] , [27] , [28] . Here, we extended the method to the growth of 2D crystals. 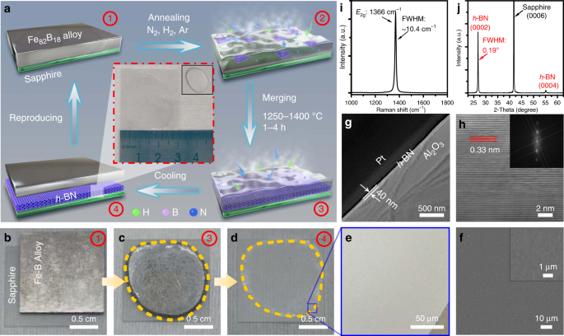Fig. 1: Fabrication of large-area multilayerh-BN on sapphire. aSchematics of multilayerh-BN grown on sapphire with Fe82B18alloy and nitrogen as reactants.b–dOM images of Fe–B alloy on sapphire before and after the growth process.e,fOM and SEM images of multilayerh-BN on sapphire.gCross-sectional TEM image of multilayerh-BN on sapphire.hHigh-resolution TEM image corresponding to (g). The fast Fourier transform (FFT) pattern is displayed in the inset.i,jTypical Raman and XRD spectra of multilayerh-BN film on sapphire. Figure 1a shows schematics of the VLSG method for multilayer h -BN growth. In the inset, our work demonstrated the reliable synthesis of large-area uniform multilayer h -BN on the surface of a 3 cm × 3 cm sapphire substrate. The current size of the h -BN films was due to the limited space and apparatus design of our CVD system only. The optical microscopy (OM) images were obtained at different stages and are presented in Fig. 1b–e (see detailed growth processes in the “Methods” section). We propose that the liquid catalyst (molten Fe 82 B 18 alloy) promoted the dissociation of N 2 , served as a solvent for B–N associate diffusion through individual atomic vacancies and assisted the nucleation and 2D lateral growth of the solid h -BN film at the liquid–solid interface. This method has the potential to scale to wafer-sizes production of high-quality multilayer h -BN, which would boost practical applications of 2D materials and their van der Waals (vdW) hetero-structures. Fig. 1: Fabrication of large-area multilayer h -BN on sapphire. a Schematics of multilayer h -BN grown on sapphire with Fe 82 B 18 alloy and nitrogen as reactants. b – d OM images of Fe–B alloy on sapphire before and after the growth process. e , f OM and SEM images of multilayer h -BN on sapphire. g Cross-sectional TEM image of multilayer h -BN on sapphire. h High-resolution TEM image corresponding to ( g ). The fast Fourier transform (FFT) pattern is displayed in the inset. i , j Typical Raman and XRD spectra of multilayer h -BN film on sapphire. Full size image VLSG of thickness-controllable multilayer h -BN on sapphire The investigation by scanning electron microscopy (SEM) verified the successful growth of a continuous and uniform h -BN film on sapphire substrate (Fig. 1f ). The cross-sectional transmission electron microscopy (TEM) image shows a typical thickness of ~40 nm and an interlayer distance of 0.33 nm (Fig. 1 g, h and Supplementary Fig. 1d ). Furthermore, the TEM images of the h -BN film suspended on a TEM grid exhibit a smooth h -BN film without any ad-layers (Supplementary Fig. 1c , e and f). Moreover, as measured by ultraviolet–visible (UV–Vis) absorption spectroscopy, the intrinsic bandgap energy of the h -BN film was ~5.9 eV (Supplementary Fig. 1a, b ), which is in agreement with previous reports [29] , [30] . The Raman spectrum of the multilayer h- BN transferred on SiO 2 (300 nm)/Si substrate exhibits the characteristic peak at 1366 cm −1 , and the full width at half maximum (FWHM) of this peak was measured to be 10.4 cm −1 , which is comparable to those of the h -BN flakes exfoliated from the h -BN crystals (Fig. 1i ). Additionally, the FWHM mapping of the E 2g mode displayed a high uniformity and low density of defects over a large area of the h -BN film (Supplementary Fig. 2 ). The X-ray diffraction (XRD) spectrum (Fig. 1j ) displays the dominant (0006) peak of the sapphire c -plane at 41.7°. In addition, the (0002) and (0004) h -BN peaks were observed at 26.6° and 55.2°, respectively, confirming that these multilayers were well aligned to the c axis that was perpendicular to the sapphire substrate [12] . The FWHM of the (0002) h -BN peak was measured to be 0.19°, indicating the highly crystalline quality of the h -BN multilayers [24] . During the VLSG method, the thickness of the h -BN can be simply controlled by adjusting the growth time and temperature. 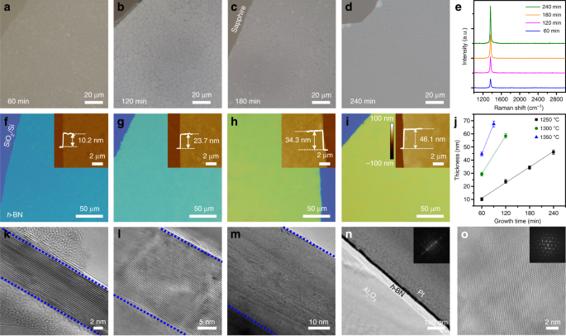Fig. 2: Controllable thickness of large-area multilayerh-BN on sapphire. a–d, Typical OM images of multilayerh-BN grown on sapphire with 60 (a), 120 (b), 180 (c) and 240 (d) minutes at 1250 °C.eCorresponding Raman spectra of multilayerh-BN with different growth times.f–iCorresponding to (a–d), multilayerh-BN are transferred onto SiO2(300 nm)/Si substrate. The inset shows the corresponding AFM images.jRelationship between growth time and thickness of multilayerh-BN. Error bars for the experimental data represent standard deviation uncertainty of thicknesses collected from different samples.k–nCorresponding TEM images of multilayerh-BN with different thicknesses.oTypical TEM image and FFT pattern (inset) of multilayerh-BN. Figure 2a–d presents typical OM images of h -BN films grown on sapphire with different growth times from 60 to 240 min at 1250 °C. Figure 2f–i shows the h -BN films (corresponding to the films in Fig. 2a–d , respectively) that were transferred onto SiO 2 (300 nm)/Si substrates. It was observed that the wrinkles caused by the mismatch of the thermal expansion coefficient between the sapphire and multilayer h -BN were completely released after the transfer. We systemically investigated the wrinkles, and the results are given in supplementary Figs. 3 – 5 . The as-transferred h -BN multilayers exhibit a homogeneous color contrast, indicating a macroscopic uniformity in their thickness. Atomic force microscopy (AFM) was further used to determine the thickness and uniformity of the h -BN films (insets in Fig. 2f–i and supplementary Figs. 6 – 8 ). The thickness of the h -BN film linearly increased according to the growth time (Fig. 2j ), and the h -BN film transferred on SiO 2 (300 nm)/Si substrate had a very smooth surface over 10 μm × 10 μm area (root-mean-square roughness ( R a ) = 0.11 nm). The Raman spectra of the transferred h -BN showed a characteristic E 2g band at 1366~1368 cm −1 using a 532 nm laser excitation (Fig. 2e ). The intensity of the E 2g band increased linearly with growth time after normalizing the intensity of characteristic silicon peak at 520 cm −1 . The well-defined layer structure of the multilayer h -BN was analysed by means of high-resolution TEM (Fig. 2k–n ). The orientation of the h -BN (0002) lattice plane was confirmed. In addition, as shown in Fig. 2o , the h- BN multilayer had highly ordered interlayer stacking. In the inset, the corresponding fast Fourier transform (FFT) pattern displays only one set of six-fold symmetric diffraction, indicating the well-defined stacking order of the as-prepared h -BN multilayers. Their stacking order was also verified via the method of H plasma treatment [31] . To control the thickness of the h -BN layers, the influence of the growth temperature was also investigated (Supplementary Fig. 9 ). The effect of the growth temperature/time on the thickness of multilayer h- BN is summarized in supplementary Table 1 . Fig. 2: Controllable thickness of large-area multilayer h -BN on sapphire. a – d , Typical OM images of multilayer h -BN grown on sapphire with 60 ( a ), 120 ( b ), 180 ( c ) and 240 ( d ) minutes at 1250 °C. e Corresponding Raman spectra of multilayer h -BN with different growth times. f – i Corresponding to ( a – d ), multilayer h -BN are transferred onto SiO 2 (300 nm)/Si substrate. The inset shows the corresponding AFM images. j Relationship between growth time and thickness of multilayer h -BN. Error bars for the experimental data represent standard deviation uncertainty of thicknesses collected from different samples. k – n Corresponding TEM images of multilayer h -BN with different thicknesses. o Typical TEM image and FFT pattern (inset) of multilayer h -BN. Full size image The epitaxial relationship between the multilayer h -BN and sapphire was suggested by cross-sectional TEM and electron backscattered diffraction (EBSD). A cross-sectional TEM image displays the interface between h -BN and sapphire (Fig. 3a ). According to the corresponding FFT patterns of the as-grown h -BN and sapphire (Fig. 3a insets), it was calculated that the [11-20] direction in the h -BN was well aligned to the [10-10] direction in the sapphire. In addition, the atomic resolution and atomic fringes in the magnified high-resolution TEM images of h -BN and sapphire also confirmed the alignment (Fig. 3b–e ). Furthermore, as shown in Fig. 3f , the pole figures of the sapphire and h -BN films proved that the alignment of the h -BN layers on sapphire was [0001] h -BN||[0001] sapphire, [10-10] h -BN||[11-20] sapphire, and [11-20] h -BN||[10-10] sapphire, consistent with previous reports [21] , [29] . Fig. 3: Epitaxial relationship between multilayer h -BN and sapphire. a High-resolution TEM image of <11-20> h -BN multilayers on sapphire along <10–10> of sapphire. The inset shows the corresponding FFT pattern from multilayer h -BN and sapphire areas, respectively. b , c TEM images with atomic resolution of multilayer h -BN ( b ) and sapphire ( c ). d , e Atomic arrangement of the h -BN layer on the sapphire substrate without rotation (R 0 ) and with a rotational angle of 30° (R 30 ). f EBSD pole figures in the (0001), (10–10), and (11–20) planes for c -plane sapphire substrate and multilayer h -BN. Full size image Mechanism of VLSG of multilayer h -BN on Fe 82 B 18 alloy To explore how B-N bonding initially forms in Fe-B alloy, we carried out in situ ambient pressure X-ray photoelectron spectroscopy (APXPS) measurements on the surface of the Fe-B alloy. The temperature-resolved evolution of the B 1s and N 1s spectra were investigated from 27 °C (300 K) to 677 °C (950 K) in a N 2 /H 2 atmosphere, which indicated the decomposition of N 2 and formation of the B-N phase on the Fe-B alloy during the heating process (Fig. 4a, b ). Here, high binding energy (BE) and low BE peak pairs, depicted as the characteristic peak of monolayer and few-layer h -BN, respectively, are centered at 190.6/397.9 eV and 189.9/397.5 eV, respectively, consistent with a previous report [14] . In addition, the B/N peak pair located at 191.4/399.4 eV was identified as a defect species [32] . With increasing temperature, the increase in the intensity ratio of the lower BE and higher BE B/N peak pairs indicates that few-layer h -BN formed gradually instead of a monolayer [14] . After annealing, the B/N atomic ratio was approximately 1, which is consistent with the multilayer h -BN synthesized at 1250 °C (Supplementary Fig. 10a–f ). Moreover, ex situ TEM and energy dispersive spectrometry (EDS) mapping of Fe and N demonstrated that layered h -BN formed at 677 °C on Fe-B nanoparticles by annealing in a N 2 /H 2 atmosphere for 6 h (Fig. 4c–f ). Fig. 4: Investigation of the h -BN growth process on Fe-B alloy. a , b B 1s ( a ) and N 1s ( b ) spectra during the in situ APXPS measurement. c , d TEM images of Fe–B nanoparticles wrapped with layered h -BN. e , f EDS mapping of Fe ( e ) and N ( f ) corresponding to ( c ). Full size image Previous studies [14] , [15] , [16] reported that N was almost completely insoluble in Cu, Ni, and Fe at 1000 °C. In this work, it was found that the Fe-B alloy played a critical role in both the decomposition of N 2 and the formation of few-layer h -BN via in situ APXPS experiments. The utilization of the Fe-B alloy broke the surface-limited growth process, which always yielded monolayer h -BN. Moreover, under a high temperature of 1250 °C, the efficiency of both the decomposition of N 2 and formation of B-N associates was improved, and then the growth rate of the multilayer h -BN increased. Time-resolved N 1s evolution at 577 °C (850 K) in a N 2 /H 2 atmosphere and growth experiments at 1250 °C for 120 min with different cooling rates were carried out the confirm the isothermal process (Supplementary Figs. 10g, h and 11 ). We propose that the abundant B in the alloy activated the isothermal segregation of the h -BN layers. In contrast to the previous growth mechanism for h -BN, the isothermal growth procedure on an active melted Fe–B alloy greatly improved the uniformity, crystallinity and smoothed surface of the h -BN layers. It may suppress the formation of thick h -BN flakes induced by cooling-induced segregation. According to the heterogeneous equilibrium in the B–Fe–N phase diagram, the N and B in the liquid comprise Fe, BN, Fe 2 B, and atomic nitrogen (details in Supplementary Figs. 12 and 13 ) [33] . The growth process at high temperatures can be divided into three stages as follows. First, the Fe-B alloy melted at 1250 °C in a N 2 atmosphere. As a precursor during this stage, the N 2 decomposed at the vapor–liquid interface and reacted with B to form chemically stable B–N associates, which was illustrated through the in situ APXPS experiments. Second, the liquid phase broke the stability of the lattice in the solid alloy and then produced enough vacancies in the lattice, which increased the diffusion of the B–N associates [34] . Crystalline h -BN structures formed at the liquid–solid interface between the molten alloy and sapphire. Finally, the B–N associates continuously diffused through the liquid and interacted with the Fe catalyst. The formation of new h -BN layers between the preformed h -BN and Fe–B alloy ensured the controllable synthesis of high-quality multilayer h -BN. The synthesis of h -BN here relied on the formation and diffusion of B–N associates during the reaction. Applications of CVD multilayer h -BN The multilayer h -BN transferred onto a SiO 2 (300 nm)/Si substrate was investigated by room-temperature Raman and photoluminescence (PL) spectroscopies for determining the optically active defect distribution [35] , [36] , [37] , [38] , [39] , [40] , [41] . As shown in supplementary Fig. 14a and b, Raman mapping of the E 2g intensity with the corresponding OM and AFM images demonstrated the uniformity of the fabricated h -BN layers. The subsequent PL intensity mapping demonstrated that optically active defects were only present at edges and wrinkles. The PL spectra at those typical spots were extracted and fitted by Lorentzian fitting (supplementary Fig. 14c ). On one hand, three peaks centered at 2.13, 1.97, and 1.81 eV are observed in the wrinkled areas, which is consistent with zero phonon line (ZPL) and corresponding one- and two-optical-phonon sidebands (PSB) [37] , [39] . These optical emissions show coincident features with a previous report, which claimed that wrinkle-induced emissions are sensitive to strain and/or local lattice symmetry distortions [39] . On the other hand, the edges of a h -BN flake on the SiO 2 (300 nm)/Si substrate show a different optical emission. The ZPL peak is located at 2.06 eV, and the corresponding PSB are evident at 1.90 and 1.74 eV. Moreover, the energy difference between the two adjacent peaks in all optical emissions is ~160 meV, which agrees well with the in-plane optical (LO/TO) phonon energy of h -BN [42] . Additionally, an overlapping multilayer h -BN on a SiO 2 (300 nm)/Si substrate was studied by Raman and PL, showing similar results (supplementary Fig. 14d–f ). The fact that no optical emissions at energies between 1.7 and 2.2 eV could be found in large uniform areas provides the possibility to artificially fabricate optically active defects for optoelectronics in the future [40] . The mechanical strength of the multilayer h -BN was investigated with AFM nanoindentation (Fig. 5a ). First, the h -BN films were transferred onto a SiO 2 (300 nm)/Si substrate patterned with circular holes. As shown in Fig. 5b , the OM image of the multilayer h -BN suspended on an array of circular holes indicates high uniformity. Subsequent AFM measurements indicated that the h -BN films were stretched tautly across the hole openings (Fig. 5c ). By indenting the free-standing film at the center of the holes, the mechanical deformation of the h -BN film was explored. Figures 5d and e present examples of the force-displacement behavior of two multilayer h -BN flakes with thicknesses of 15.7 and 32.6 nm that were lying on circular holes with diameters of 1.6 and 2.2 μm, respectively. The Young’s modulus of the multilayer h -BN flakes was derived by fitting the force-displacement curves [16] , [43] . We measured 30 positions for each piece of h -BN flake in the uniform thickness, and the distribution of the derived values was plotted in Fig. 5f . The values of Young’s modulus were approximately 1.04 ± 0.1 TPa, which agrees within experimental error with the theoretical value [12] , [16] . The results indicated that the high mechanical strength of these multilayer h -BN films was independent of their thickness. Fig. 5: Mechanical strength of multilayer h -BN film and electron transport of the h -BN/graphene/ h -BN device. a Schematic of nanoindentation on suspended multilayer h -BN film. b OM image of h -BN membranes lying on SiO 2 (300 nm)/Si substrate with patterned circular wells. c AFM image of one membrane, 2.2 μm in diameter. The solid line is a height profile along the dashed line. d Measured force-displacement curves of multilayer h -BN with different thicknesses. e Measured force-displacement curves of multilayer h -BN with different film diameters. f Histogram of Young’s modulus with different thicknesses. Dashed lines represent Gaussian fits to data. g Schematic diagram of the h -BN/graphene/ h -BN Hall bar configuration. h The relationship of R xx and R xy versus gate voltage ( V g ) at 300 K under 1 T. An OM image of the h -BN/graphene/ h -BN Hall bar device is shown in the inset. i Magnetic field dependence of the carrier mobility versus V g . j Normalized magneto-conductivity (MC) measured at different temperatures with V g at approximately −40 V; those solid lines are fitting curves. k Temperature dependence of three characteristic lengths (L φ, L i, L ∗ ) extracted from ( j ). l Normalized MC measured at low temperatures with V g maintained at 15 V. m Temperature dependence of L φ, L i and L ∗ extracted from ( l ). Error bars in ( k ) and ( m ) for the experimental data represent standard deviation of uncertainty in characteristic lengths (L φ , L i, L ∗ ) extraction. Full size image To evaluate the applicability of the multilayer h -BN as a dielectric, graphene sandwiched between multilayer h- BN films was patterned into a Hall bar configuration, and the electronic performance of graphene was evaluated (Fig. 5g ). The longitudinal resistance ( R xx ) and transversal resistance ( R xy ) of the device were measured under 1 T at 27 ° C (300 K), and the OM image of the device is shown in the inset (Fig. 5h ). The carrier mobility of graphene at 27 ° C (300 K) under different magnetic fields, extracted by μ = 1/ B ∙( R xy ∙ L )/ ( R xx ∙ W ) [1] , was in the range of 0.5~1 m 2 V −1 s −1 (Fig. 5i ). As a baseline, the carrier mobility of CVD-grown graphene transferred onto SiO 2 (300 nm)/Si substrate was just slightly higher than 0.3 m 2 V −1 s −1 (Supplementary Fig. 16 ). Direct growth of graphene on h -BN [44] or cleaner transfer of graphene [45] could achieve better performance of field effect devices. Furthermore, the magneto-conductivity (MC) was measured at low temperatures with different back-gate biases ( V g ) to investigate the weak localization (WL) and weak anti-localization (WAL) phenomenon of graphene (Fig. 5j–m ). For this study, we used the expression for the WL-induced conductivity correction as theoretically suggested with three parameters: the phase coherence length ( L φ ), elastic intervalley scattering length ( L i ) and intravalley scattering length ( L * ) [46] . When V g was at −40 V, a positive MC was collected, which clearly presented the WL effect (Fig. 5j ). Both intravalley and intervalley scattering were strong, such that L φ ≫ L i ≳ L * (Fig. 5k ). However, when V g was fixed at approximately 15 V, the WL was transformed into WAL with increasing temperature (Fig. 5l ). In addition, L φ < L i , L * (Fig. 5m ). Overall, the distance of each of two defects in the h -BN was larger than the length of the scattering (approximately 400 nm), which was comparable to that in a previous report [47] . In summary, high-quality multilayer h- BN with a controllable thickness was achieved on sapphire via the VLSG method. The use of molten Fe 82 B 18 enabled the uniform isothermal segregation of multilayer h -BN with a thickness of 5~50 nm. The 2D growth was strictly limited to the interface between the liquid Fe 82 B 18 and the sapphire substrate. The in situ APXPS helped us to observe how the B-N associates initially formed and understand the associated segregation mechanism. The existence of vacancies in the liquid alloy increased the diffusion of the B-N associates and then accumulated the multilayer h -BN formed at high temperature. Moreover, the PL, Raman, AFM nano-indentation and electron transport measurements provided evidence for the fabrication of high-quality multilayer h- BN. The VLSG method demonstrated an efficient method for the synthesis of h -BN. The approach exhibited potential for large-area synthesis of multilayer h -BN and integration of other 2D materials. Fabrication of Fe 82 B 18 alloy Following the Fe-B binary phase diagram, Fe 2 B and Fe were chosen as initial reactants, and the molar ratio between Fe 2 B and Fe was set as 1:2.3. The raw materials were mixed thoroughly and annealed at 1500 °C for 120 min. Then, the samples were cooled naturally. 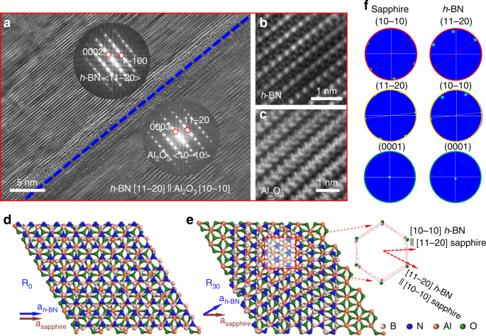Fig. 3: Epitaxial relationship between multilayerh-BN and sapphire. aHigh-resolution TEM image of <11-20>h-BN multilayers on sapphire along <10–10> of sapphire. The inset shows the corresponding FFT pattern from multilayerh-BN and sapphire areas, respectively.b,cTEM images with atomic resolution of multilayerh-BN (b) and sapphire (c).d,eAtomic arrangement of theh-BN layer on the sapphire substrate without rotation (R0) and with a rotational angle of 30° (R30).fEBSD pole figures in the (0001), (10–10), and (11–20) planes forc-plane sapphire substrate and multilayerh-BN. The whole process was maintained at ambient pressure under Ar flows. Synthesis of multilayer h- BN on sapphire Multilayer h- BN was synthesized on sapphire with a (0001) facet under ambient pressure by using an Fe 82 B 18 alloy and N 2 as reactants. First, a plate of Fe-B alloy was placed on top of the sapphire and loaded into the reaction chamber. The system was annealed at 1,250 °C for 60 min under a mixed Ar/H 2 (300/50 sccm) ambient atmosphere. Then, N 2 was introduced with a flux of 300 sccm at 1250 °C for 60 min. The h -BN multilayer isothermally segregated on the interface between the sapphire and Fe-B alloy. Finally, the reaction chamber cooled to room temperature at a rate of 10 °C/min under a mixed Ar/H 2 (300/50 sccm) gas. The Fe–B alloy could be easily peeled off and left the h -BN multilayer on the sapphire substrate. h -BN Characterizations Surface morphology and crystalline properties of the h -BN layers were investigated by SEM (Zeiss supra55, operated at 1.5 kV), AFM (Bruker Dimension Icon, tapping mode) and XRD (Bruker D8 DISCOVER). TEM (JEM-2100F, operated at 200 kV), PL & Raman spectroscopy (WITec Alpha 300 R, 532 nm laser with ×50 objective lens, operated at room temperature) and UV–Vis absorption spectroscopy (Agilent EV 300) evaluates the quality of as-synthesized multilayer h -BN preliminarily. In situ XRD (Bruker D8 ADVANCE) and APXPS (Species, Al Kα) were used to understand the phase transition in Fe-B alloy and the growth mechanism of multilayer h -BN. TEM (JEM-ARM 300 F, operated at 80 kV), focused ion beam (FIB, Helios Nanolab 600) and EBSD (Bruker e − Flash FS ) were employed to understand the epitaxial relationship between multilayer h -BN and sapphire substrate. For mechanical characterizations, a diamond-coated AFM tips (Tap190DLC, Budget sensors) was used and the spring constant of the AFM cantilever was calibrated as 75.4 N m −1 . In situ APXPS and XRD characterization For in situ APXPS measurements, the Fe 82 B 18 alloy was cleaned by Ar+ sputtering to remove surface residues. During the heating process, a N 2 /H 2 (3:1) mixed gas was introduced into the chamber, and the pressure was kept at 1 mbar constantly. 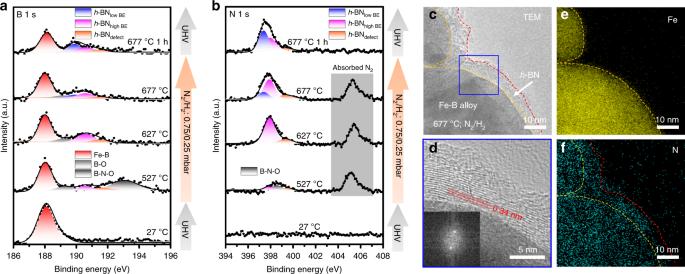Fig. 4: Investigation of theh-BN growth process on Fe-B alloy. a,bB 1s (a) and N 1s (b) spectra during the in situ APXPS measurement.c,dTEM images of Fe–B nanoparticles wrapped with layeredh-BN.e,fEDS mapping of Fe (e) and N (f) corresponding to (c). 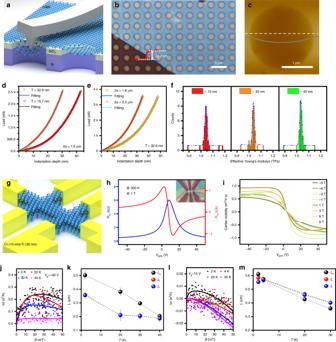Fig. 5: Mechanical strength of multilayerh-BN film and electron transport of theh-BN/graphene/h-BN device. aSchematic of nanoindentation on suspended multilayerh-BN film.bOM image ofh-BN membranes lying on SiO2(300 nm)/Si substrate with patterned circular wells.cAFM image of one membrane, 2.2 μm in diameter. The solid line is a height profile along the dashed line.dMeasured force-displacement curves of multilayerh-BN with different thicknesses.eMeasured force-displacement curves of multilayerh-BN with different film diameters.fHistogram of Young’s modulus with different thicknesses. Dashed lines represent Gaussian fits to data.gSchematic diagram of theh-BN/graphene/h-BN Hall bar configuration.hThe relationship ofRxxandRxyversus gate voltage (Vg) at 300 K under 1 T. An OM image of theh-BN/graphene/h-BN Hall bar device is shown in the inset.iMagnetic field dependence of the carrier mobility versusVg.jNormalized magneto-conductivity (MC) measured at different temperatures withVgat approximately −40 V; those solid lines are fitting curves.kTemperature dependence of three characteristic lengths (Lφ,Li,L∗) extracted from (j).lNormalized MC measured at low temperatures withVgmaintained at 15 V.mTemperature dependence of Lφ,Liand L∗extracted from (l). Error bars in (k) and (m) for the experimental data represent standard deviation of uncertainty in characteristic lengths (Lφ, Li,L∗)extraction. When the temperature reached the set point, the N 1s spectrum and B 1s spectrum were collected. Finally, the Fe 82 B 18 alloy was cooled to room temperature naturally. For in situ XRD measurements, the XRD spectra of the original Fe–B alloy were measured in advance for further comparison. First, N 2 (400 sccm) was introduced into the chamber at ambient atmosphere and flowed during the whole process. Then, the stage began to heat at a heating rate of 10 °C min −1 . When the temperature reached the set point, the measurement process consumed ~30 min for each calibration. After that, the system was cooled down at a rate of 10 °C min −1 . Two additional temperature spots were calibrated during the cooling process. Finally, the Fe–B alloy was cooled to room temperature naturally. Electronic device fabrication The h -BN/graphene/ h -BN van der Waals (vdW) hetero-structure was assembled by the “peel and stack” technique. To fabricate the hetero-structure, we started with as-transferred monolayer graphene on top of an oxidized Si wafer. The monolayer graphene was synthesized via CVD method and the growth process had been reported in earlier literature [48] . The graphene monolayer was picked up by h -BN multilayer attached to a PDMS/PPC membrane and then stacked on to another freshly cleaved h -BN film that was grown. The detailed procedures illustrated graphically in Supplementary Fig. 15 . The “peel and stack” technique ensured a clean interface between the flakes. Then, the hetero-structure was shaped into a Hall bar with a channel length of 4 μm and a width of 2 μm. After that, magnetron sputtered Cr (15 nm)/Ti (30 nm) defined multiple electrodes for transport measurement.